RETRACTED ARTICLE: Ornithine-A urea cycle metabolite enhances autophagy and controlsMycobacterium tuberculosisinfection Macrophages are professional phagocytes known to play a vital role in controlling Mycobacterium tuberculosis ( Mtb ) infection and disease progression. Here we compare Mtb growth in mouse alveolar (AMs), peritoneal (PMs), and liver (Kupffer cells; KCs) macrophages and in bone marrow-derived monocytes (BDMs). KCs restrict Mtb growth more efficiently than all other macrophages and monocytes despite equivalent infections through enhanced autophagy. A metabolomics comparison of Mtb -infected macrophages indicates that ornithine and imidazole are two top-scoring metabolites in Mtb -infected KCs and that acetylcholine is the top-scoring in Mtb -infected AMs. Ornithine, imidazole and atropine (acetylcholine inhibitor) inhibit Mtb growth in AMs. Ornithine enhances AMPK mediated autophagy whereas imidazole directly kills Mtb by reducing cytochrome P450 activity. Intranasal delivery of ornithine or imidazole or the two together restricts Mtb growth. Our study demonstrates that the metabolic differences between Mtb -infected AMs and KCs lead to differences in the restriction of Mtb growth. Alveolar macrophages (AMs) are the first cells that come into contact with Mycobacterium tuberculosis ( Mtb ) in the lung, but cannot completely eliminate it, thus serving as Mtb niches. Despite effective host defense strategies, Mtb manages to escape from phagosome-lysosome fusion and other antimicrobial defense mechanisms and thus, actively replicates in AMs and survives inside phagosomes [1] . Depletion of AMs in vivo attenuates Mtb growth in the lungs because the environment for intracellular replication and immune evasion is destroyed [2] . Therefore, it is important to understand why AMs are less efficient than other macrophages in Mtb clearance. In addition to the lungs, which are the primary organ of infection, Mtb bacilli can spread to extra-pulmonary sites among which the liver is the least frequently infected organ representing <1% of all tuberculosis (TB) infections [3] . Liver macrophages (Kupffer cells; KCs) are highly phagocytic, reside within the lumen of liver sinusoids, and protect the liver from gut-derived toxic materials and bacterial infections [4] . KCs can control Mtb growth, and thus rendering the liver an unfavorable site for mycobacterial colonization [5] . However, it is not clear how KCs eliminate mycobacterial infections more efficiently than other macrophage populations. Thus, identification of these mechanisms would facilitate the development of immunomodulatory strategies to boost AM-mediated immunity to Mtb and to prevent progression from latent TB infection to the active disease state. In the current study, we compare Mtb growth in AMs, peritoneal macrophages (PMs), bone marrow-derived monocytes (BDMs) and KCs. We also identify mechanisms involved in the enhanced restriction of Mtb growth in KCs compared with AMs and PMs. KCs restrict Mtb growth better than AMs, PMs and BDMs We compared Mtb H37Rv growth in AMs, PMs, KCs and BDMs. Both monocyte and macrophage populations demonstrated similar numbers of bacteria at 2 h post-infection (Fig. 1 ). However, at day 5 post-infection, AMs, PMs and BDMs had 3-fold, 2.5-fold and 2-fold higher Mtb than KCs indicating that KCs are more efficient than AMs, PMs and BDMs in inhibiting Mtb growth. Fig. 1: KCs restrict Mtb growth better than AMs, PMs and BDMs. Alveolar (AMs), peritoneal (PMs) and liver macrophages (KCs) as well as bone marrow-derived monocytes (BDMs) from C57BL/6 mice were isolated and infected with Mtb H37Rv at an MOI of 1:2.5 (1 AM, PM, KC, BDMs and 2.5 Mtb ). Intracellular CFUs were demonstrated 2 h and 5 days post-infection. Statistical analysis was performed with paired two-tailed t test and mean ± SDs are shown. p < 0.0003, p < 0.0001, p < 0.0015, ns: not significant. The data shown are the average of five independent experiments. Full size image Mtb induces equal cytokine levels and apoptosis in KCs, AMs and PMs We speculated that the Mtb resistance to KCs caused by the ability of these cells to produce more cytokines. There were no significant differences in cytokine production among Mtb -infected AMs, PMs and KCs (Fig. 2a–d ) suggesting that the difference in growth restriction is not attributable to cytokine production. Fig. 2: Mtb induces equal cytokine levels and apoptosis in KCs, AMs and PMs. AMs, PMs and KCs from C57BL/6 mice were isolated and infected with Mtb H37Rv as mentioned in Fig. 1 , and after 72 h, the ( a ) TNF-α. p < 0.0048 ( b ) IL-1β. p < 0.0241, p < 0.014 ( c ) IL-6 and ( d ) IL-10 cytokines levels in culture supernatants were measured by ELISA. p < 0.0144, p < 0.0129, p < 0.0077; ns not significant ( e , f ) AMs, PMs and KCs were also cultured with gamma-irradiated Mtb (γ- Mtb ) for 24 h. e TLR-2. p < 0.0011, p < 0.0011 and f TLR-4 expression was demonstrated by flow cytometry. p < 0.0011. AMs, PMs, and KCs were infected with Mtb H37Rv and after 72 h, g iNOS and h Arg-1 mRNA expression was demonstrated by real-time PCR. The mean ± SD of the fold change in mRNA levels in infected macrophages compared to uninfected macrophages is represented. AMs, PMs and KCs from C57BL/6 mice were isolated and infected with Mtb H37Rv at an MOI of 1:2.5. After 72 h, apoptosis was demonstrated by the Phosphatidyl-serine exposure assay/Annexin-V/PI staining and confirmed by the TUNEL assay. i The percentage of the early phase apoptotic cells is shown. p < 0.0031, p < 0.0041. j A representative flow cytometry plot for the TUNEL assay. k The percentage of the late phase apoptotic cells is shown. p < 0.0033, p < 0.0013, ns: not significant. Statistical analysis was performed with paired two-tailed t test and presented as mean ± SD. Data represent the average of five independent experiments. Full size image TLR-2 and TLR-4 play important roles during Mtb infection, and are expressed differentially in the various populations of macrophages [6] . There was no significant difference in TLR-2 and TLR-4 expression among AMs, PMs and KCs cultured with γ- Mtb (10 µg/ml), as demonstrated using flow cytometry (Fig. 2e, f ). Moreover, there was no significant difference in iNOS and Arg-1 gene expression among Mtb H37Rv-infected AMs, PMs and KCs (Fig. 2g, h ). Mtb -infected macrophages initiate a respiratory burst and produce higher levels of reactive oxygen species (ROS), critical for the bactericidal effect [7] . We evaluated the intracellular ROS production and found no difference among AMs, PMs and KCs 24 h after Mtb infection using flow cytometry (Supplementary Fig. 2a, b ) indicating that ROS is not involved in Mtb growth inhibition. Further, we monitored nitric oxide (NO) levels in these macrophages as NO is one of the major limiting factors regarding Mtb growth and function [8] . We measured the nitrate (NO 3 − ) and nitrite (NO 2 – ) produced from NO released into culture supernatants 72 h after Mtb infection. Mtb -infected KCs were lower NO producers than Mtb -infected AMs and PMs suggesting that reduced Mtb growth in KCs is not mediated through NO-dependent killing (supplementary Fig. 2c ). Conversely, another study also showed that enhanced Arg-1 activity involved in controlling TB [9] . Therefore, we measured the conversion of arginine to ornithine in cell lysates after 72 h of Mtb infection and found higher arginase activity in Mtb -infected KCs compared with Mtb -infected AMs and PMs (Supplementary Fig. 2d ). Apoptosis is one of the major host defense mechanisms used by macrophages to restrict Mtb growth [10] . There was no significant difference in the Annexin V + (apoptotic) levels among Mtb -infected AMs, PMs and KCs (Fig. 2i ). Similar results were obtained in complementary experiments performed to examine DNA fragmentation (TUNEL assay) in late-phase apoptotic cells (Fig. 2j, k ). The viability of AMs, PMs and KCs was similar after Mtb infection (Supplementary Fig. 3 ). Kupffer cell autophagy is increased by Mtb infection The above findings demonstrate that the differences in Mtb growth restriction by AMs, PMs and KCs were not due to differences in inflammatory cytokine production, TLR expression, ROS or NO production or apoptosis. Autophagy is another vital defense mechanism activated in response to nutrient starvation or by metabolic, physiological, pharmacological and immunological means which in turn involved in antimicrobial defense mechanisms [11] . To examine whether autophagy differs in Mtb -infected mouse AMs, PMs and KCs, all groups of macrophages were infected with Mtb . LC-3 (a widely used specific marker of autophagy) expression was evaluated at 3dpi by flow cytometry. The mean fluorescence intensity of LC-3 + Mtb -infected KCs was significantly higher than that of LC-3 + Mtb -infected AMs and PMs (Fig. 3a, b ), whereas no significant difference was observed between Mtb -infected AMs and PMs. Rapamycin was used as a positive control. Fig. 3: Kupffer cell autophagy is increased by Mtb infection. AMs, PMs, and KCs from C57BL/6 mice were infected with Mtb H37Rv. After 72 h, LC-3 positive cells were evaluated by flow cytometry. a Representative flow cytometry plot for LC-3. b Mean fluorescence intensity (MFI) of LC-3 expression. n = 3 experiments. p < 0.0024, p < 0.0064, p < 0.0051, p < 0.0058. c Total protein was extracted from the above cells and western blotting was performed. A representative blot depicting the levels of LC-3 and p62/SQSTM1 in the control, Mtb H37Rv-infected and bafilomycin A1 treated macrophages is shown. GAPDH was used as a loading control. d Normalized fold intensities of LC-3B, p62 levels in Mtb H37Rv-infected macrophages relative to the levels in the uninfected control. n = 3 experiments. p < 0.0098, p < 0.0263, p < 0.028. e A representative micrograph of LC3-B, ATG-7, ATG-5 and Beclin-1 in AMs and KCs. Blue: DAPI; green: LC-3B and ATG-7; red: ATG-5 and Beclin-1. Images of multiple fields were taken at 63× magnification with oil immersion. f The number of LC-3B puncta relative to the cell area was measured using ImageJ and quantified in 10 cells per condition. g Macrophages were labeled with an autophagy sensor expressing RFP-GFP-LC3B for 48 h. The labeled macrophages were then infected with Mtb H37Rv for 72 h. The cells were fixed, and LC-3B was analyzed by confocal microscopy. Autophagosomes show both GFP (green) and RFP (red) signals. Autophagosome-lysosome fusion results in RFP-positive and GFP-negative dots. Scale bars: 5 µm. h Quantification of the number of LC-3B positive autophagosomes (yellow fluorescence) and autolysosomes (red fluorescence) in control, Mtb -infected macrophages followed by treatment with or without chloroquine is shown. n = 3 experiments. p < 0.0142, p < 0.0025, p < 0.0063, p < 0.0047. i KCs from C57BL/6 mice were isolated and transfected with siRNAs targeting LC-3B, ATG-5, ATG-7 and Beclin-1 or with control siRNA and then infected with Mtb H37Rv. After 5 days, CFUs were counted. n = 5 experiments. Data are presented as the mean ± SD using paired two-tailed t test. Full size image We confirmed these findings by western blotting as Mtb -infected KCs expressed LC-3B at higher levels compared with Mtb -infected AMs. In contrast, Mtb -infected KCs expressed reduced levels of autophagy substrate p62/SQSTM1 than Mtb -infected AMs (Fig. 3c, d ) suggesting impairment of autophagy-dependent degradative activity in AMs and PMs. In addition, Mtb induced LC-3B levels were further increased by treatment with the vacuolar H + -ATPase inhibitor, bafilomycin A1 (baf A1), indicating a real autophagic flux in KCs (Fig. 3c, d ) whereas Mtb -infected AMs showed reduced levels of LC-3B and did not respond to baf A1 treatment suggesting suppressed autophagy. We also evaluated the levels of ATG-5, ATG-7 and Beclin-1 proteins (Supplementary Fig. 4a, b ), which are autophagy regulators. PMs were equal or less autophagic compared with AMs. We further confirmed that Mtb -infected AMs and PMs compared with Mtb -infected KCs expressed higher levels of LC-3B, ATG-5, ATG-7 and Beclin-1 mRNAs (Supplementary Fig. 4c ) by real-time PCR (RT-PCR). In addition, confocal microscopy imaging revealed increased expression of ATG-5, ATG-7 and Beclin-1 and markedly enhanced LC-3B puncta formation in Mtb -infected KCs vs. Mtb -infected AMs and PMs (Fig. 3e, f ). The mean immunofluorescence intensities of LC-3B, ATG-5, ATG-7 and Beclin-1 were significantly higher in Mtb -infected KCs vs. Mtb- infected AMs and PMs (Supplementary Fig. 5 ). To examine further the functional role of KCs in generating autophagy flux during Mtb infection, we labeled AMs, PMs and KCs with an autophagy sensor expressing RFP-GFP-LC-3B to monitor LC-3B accumulation in autophagosomes and autolysosomes. In pH neutral autophagosomes, RFP-GFP-LC-3B produces a yellow signal, while the sensor produces a stronger red fluorescence signal in autolysosomes due to loss of the pH sensitive GFP signal. In KCs infected with Mtb , autophagy flux was associated with increased autolysosome (red fluorescence) numbers (Fig. 3g, h ). In contrast, in AMs infected with Mtb , the autophagosomes (yellow fluorescence) showed a failure to fuse with lysosomes indicating suppressed autophagy (Fig. 3g, h ). Furthermore, chloroquine treatment of Mtb -infected KCs and AMs inhibited autolysosome fusion. Autophagy increases restriction of Mtb growth To examine whether increased autophagy in KCs is related to the enhanced clearance of Mtb , AMs and KCs were transfected with siRNAs to LC-3B, ATG-5, ATG-7, Beclin-1 and with control siRNA and Mtb growth was demonstrated. The transfection efficiency of siRNAs as quantified by western blot was >85% (Supplementary Fig. 6 ). At 5 days post infection, Mtb growth was significantly enhanced in KCs transfected with LC-3B, ATG-5, ATG-7 and Beclin-1 siRNAs compared with KCs transfected with control siRNA (Fig. 3i ). Similarly, significant but marginal increases in Mtb burden were noted in AMs and PMs transfected with LC-3B, ATG-5, ATG-7 and Beclin-1 siRNAs compared with control siRNA transfected cells (Supplementary Fig. 7 ). Metabolic profiles of Mtb -infected AMs and KCs Because liver cells are metabolically active compared with various other cell types, and autophagy can regulate metabolic changes [12] , we asked whether Mtb -infected AMs and KCs differed in their metabolic activity. Mouse AMs and KCs were isolated and infected with Mtb H37Rv. After 72 h, the control and Mtb -infected cell lysates were analyzed by liquid chromatography-mass spectrometry (LC-MS). Using supervised partial least squares discriminant analysis (PLS-DA), we found that most of the data were within the 95% confidence region. The metabolites in the four groups were closely related to each other (Supplementary Fig. 8a ). There was a minor overlap between the control and infected AMs (Fig. 4a ), whereas a high level of segregation was noted between the control and infected KCs and between the infected AMs and infected KCs (Fig. 4b, c ), representing a significant metabolite difference between the groups. Seventy-five metabolites were identified and a graphical representation of the individual metabolite levels in AMs and KCs is provided as a heat map (Supplementary Fig. 8b ), showing the relative concentration of the metabolites (increase and decrease) in Mtb infection across different groups. Among the segregated groups, using the variable importance in the projection (VIP) score, we identified 25 metabolites with VIP scores >1.0 (considered to be the most significant metabolites) between the control and Mtb H37Rv-infected AMs or KCs as the most important in the group segregation (Fig. 4d ). Quantitative metabolite enrichment analysis was performed, and the metabolic pathways of 25 metabolites were represented (Fig. 4e ). All significant metabolites were mapped to the biological pathways in the Kyoto encyclopedia of genes and genomes database, ultimately identifying 20 pathways. The results indicated that three and eight pathways were involved in Mtb H37Rv-infected AMs and KCs, respectively. 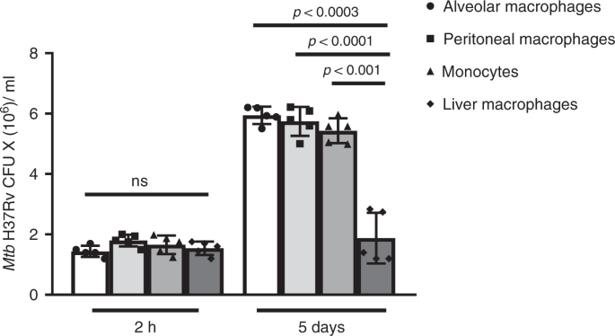Fig. 1: KCs restrictMtbgrowth better than AMs, PMs and BDMs. Alveolar (AMs), peritoneal (PMs) and liver macrophages (KCs) as well as bone marrow-derived monocytes (BDMs) from C57BL/6 mice were isolated and infected withMtbH37Rv at an MOI of 1:2.5 (1 AM, PM, KC, BDMs and 2.5Mtb). Intracellular CFUs were demonstrated 2 h and 5 days post-infection. Statistical analysis was performed with paired two-tailed t test and mean ± SDs are shown.p< 0.0003,p< 0.0001,p< 0.0015, ns: not significant. The data shown are the average of five independent experiments. Among them, three specific pathways were involved in both Mtb H37Rv-infected AMs and KCs (Supplemental Table 1 ). Furthermore, we selected the metabolites with the highest VIP scores as the most significant in the segregation of metabolic changes. Of these, two metabolites, ornithine (VIP = 1.8) and imidazole (VIP = 1.6) were elevated in infected KCs and one metabolite, acetylcholine (VIP score = 2.8) was elevated in the infected AMs. Besides identifying metabolic profiles in AMs and KCs, we quantified the levels of ornithine and imidazole in AMs, PMs, BDMs and KCs. At 72 h after Mtb infection, AMs, PMs and BDMs expressed lower levels of ornithine and imidazole compared with Mtb -infected KCs (Supplementary Fig. 9 ). IL-4 treated macrophages were used as positive control for ornithine production. Fig. 4: Metabolic profiles of Mtb -infected AMs and KCs. AMs and KCs from C57BL/6 mice were isolated and infected with Mtb H37Rv. After 72 h, cell lysates were analyzed using LC-MS. A representative score plot of the partial least squares discriminant analysis (PLS-DA) was generated using MetaboAnalyst. PLS-DA models were validated using R 2 and Q 2 based on LOOCV (leave one out cross-validation); the four-component model was selected as the optimized model with R 2 = 0.95 and Q 2 = 0.58. The significance of the model was demonstrated by a permutation test with 100 testing iterations using a separation distance of p < 0.01. a AMs control (red); AMs Mtb H37Rv (green). b KCs control (red); KCs Mtb H37Rv (green). c AMs Mtb H37Rv (red); KCs Mtb H37Rv (green). d Representation of 25 metabolites with VIP (variable importance of projection) scores greater than 1.0 based on PLS-DA considered significant. On the extreme right, red and green indicates high and low levels of metabolites, respectively. e Quantitative metabolite sets enrichment overview using metabolite set enrichment analysis (MSEA) with the fold change showing the metabolic pathways of 25 metabolites selected based on their VIP scores greater than 1. The arrow indicates upregulated metabolites and pathways in Mtb H37Rv-infected KCs. f KCs from C57BL/6 mice were isolated and infected with Mtb H37Rv at an MOI of 1:2.5 (1 AM and 2.5 Mtb ). At 2 h post-infection, nor-NOHA were added at indicated concentrations. Intracellular CFUs were demonstrated 5 days post-infection. Statistical analysis was performed with paired two-tailed t test and presented as mean ± SD. Data shown are representative of five independent experiments. Full size image To confirm that KCs restricted Mtb growth due to the presence of high levels of ornithine, we infected KCs with Mtb H37Rv and added nor-NOHA (arginase inhibitor that blocks ornithine production) at 10 µM to some cultured cells. Treatment with nor-NOHA significantly enhanced Mtb growth in KCs compared with no treatment control (Fig. 4f ). Moreover, treatment of Mtb -infected KCs with nor-NOHA significantly downregulated LC-3B and autophagy-relevant genes (Supplementary Fig. 12 ). Ornithine, imidazole and atropine affect Mtb growth Because ornithine and imidazole were expressed in Mtb -infected AMs at lower levels than in Mtb -infected KCs, we demonstrated the effect of ornithine and imidazole on Mtb growth in AMs. Treatment with both ornithine and imidazole significantly inhibited Mtb growth in AMs at 10 mM concentration than in the untreated cells (Fig. 5a ). This level was further reduced when Mtb -infected AMs were treated with ornithine and imidazole together (5 mM each) which approximates rapamycin-induced growth restriction (Fig. 5b ). Fig. 5: Ornithine, imidazole and atropine affect Mtb growth. AMs were infected with Mtb H37Rv. At 2 h post-infection, ornithine and imidazole alone or in combination were added alongside atropine. Intracellular CFUs were demonstrated after 5 days post-infection. a Ornithine and imidazole alone, b in combination of both, c atropine. p < 0.0181, p < 0.0112. n = 5 experiments each. d A representative micrograph of LC3-B, ATG-7, ATG-5 and Beclin-1 in AMs and KCs. Blue: DAPI; green: LC-3B and ATG-7; red: ATG-5 and Beclin-1. Images of multiple fields at 63× magnification were taken with oil immersion. e The number of LC-3B puncta relative to the cell area (10 cells per condition) was quantified using ImageJ. Data shown are representative of five independent experiments. f Total protein was extracted and western blotting was performed. A representative blot depicting the levels of LC-3 and p62/SQSTM1 in the control and Mtb -infected macrophages followed by treatment with ornithine and imidazole is shown. GAPDH was used as a loading control. g Normalized fold intensities of LC-3B and p62 levels in Mtb -infected and ornithine or imidazole treated macrophages compared with the levels in the uninfected control. p < 0.0072, p < 0.019, ns not significant. n = 3 experiments. h Alveolar macrophages were labeled with an autophagy sensor expressing RFP-GFP-LC3B for 48 h. Macrophages were then infected with Mtb followed by treatment with ornithine or imidazole for 72 h. Cells were fixed, and LC-3 was analyzed by confocal microscopy. Scale bars: 5 µm. i Quantification of the number of LC-3B positive autophagosomes (yellow fluorescence) and autolysosomes (red fluorescence) in control and Mtb -infected macrophages treated with ornithine and imidazole. p < 0.0041, p < 0.0034. n = 3 experiments. j AMs from C57BL/6 mice were isolated and transfected with the siRNAs targeting LC-3B, ATG-5, ATG-7 and Beclin-1 or with control siRNA, infected with Mtb and then treated with 10 mM ornithine. After 5 days, CFUs were counted. p < 0.0097, p < 0.0067, p < 0.046, p < 0.0327. n = 5 experiments. Data are presented as the mean ± SD using paired two-tailed t test. Full size image We found elevated levels of acetylcholine (Ach) in Mtb- infected AMs (Fig. 4d ). Therefore, we examined the effect of inhibiting acetylcholine by atropine, an acetyl choline antagonist on Mtb growth. Atropine treatment significantly inhibited Mtb growth in AMs at 1, 5 and 10 mM compared with the untreated control (Fig. 5c ). Ornithine increases autophagy in Mtb -infected AMs We asked whether ornithine and imidazole enhance autophagy. Treatment with ornithine upregulated LC-3B, ATG-5, ATG-7 and Beclin-1 (Fig. 5d ), suggesting that ornithine treatment enhances autophagy in Mtb -infected macrophages in a concentration-dependent manner as demonstrated by confocal microscopy. We also observed distinctly enhanced LC-3B puncta formation (Fig. 5e ) in Mtb -infected AMs treated with ornithine. In contrast, imidazole had no effect on autophagy in Mtb -infected AMs (Fig. 5d ). The mean immunofluorescence intensities for LC-3B, ATG-5, ATG-7 and Beclin-1 were significantly higher in Mtb -infected AMs treated with ornithine than in Mtb- infected AMs treated with imidazole (Supplementary Fig. 10 ). Additionally, ornithine treated Mtb -infected AMs exhibited increased levels of LC-3B and reduced levels of p62 compared with imidazole treated Mtb -infected AMs as demonstrated by western blotting (Fig. 5f, g ). Moreover, ornithine treatment induced LC-3B levels were further increased by treatment with baf A1, indicating a real autophagic flux in ornithine treated Mtb -infected AMs. In this experiment, we used a fluorescently labeled autophagy sensor to confirm that ornithine triggered genuine autophagic flux, associated with increased autolysosomal (red fluorescence) accumulation (Fig. 5h, i ). Taken together, these findings demonstrated that ornithine treatment triggers autophagy in AMs. Next, we asked whether ornithine-dependent enhanced autophagy was involved in Mtb clearance. Ornithine (10 mM) significantly inhibited Mtb growth in AMs 5 days post-infection as observed previously (Fig. 5j ). However, siRNAs to LC-3B, ATG-5, ATG-7 and Beclin-1 significantly eliminated the ornithine-dependent Mtb growth inhibition in AMs compared with the control siRNA suggesting that ornithine inhibits Mtb growth by enhancing autophagy. Ornithine limits ammonia and activates AMPK Ammonia (NH 3 ) is produced in cells through deamination of amino acids. Mtb also produces ammonia in infected macrophages, which is detrimental to macrophages and enhances Mtb growth [13] . Ornithine converts excess ammonia to urea in the liver [14] . Since we found Mtb -infected KCs produced significantly higher levels of ornithine compared with Mtb -infected AMs, we asked whether reduced ammonia levels by ornithine in Mtb -infected KCs had any effect on autophagy and Mtb growth. At 72 h after infection, AMs produced significantly higher levels of ammonia (NH 4 + /NH 3 ) than KCs (Fig. 6a ). Treatment of Mtb -infected AMs with ornithine reduced the ammonia levels to a level similar to that of Mtb -infected KCs. Conversely, treatment of Mtb -infected KCs with 10 µM nor-NOHA increased ammonia levels (Fig. 6a ). Fig. 6: Ornithine limits ammonia and activates AMPK. AMs and KCs from C57BL/6 mice were isolated and infected with Mtb H37Rv at an MOI of 1:2.5. After 72 h. a NH 4 + /NH 3 levels were measured in the cell lysates treated with ornithine or nor-NOHA (arginase inhibitor) by spectrophotometric analysis at 570 nm with extrapolation from the standard curve and expressed in nmol (mean ± SD). Data are representatives of five independent experiments. b A representative micrograph of LC3-B, ATG-7, ATG-5 and Beclin-1 in AMs treated with ornithine or NH 4 Cl and KCs treated with NH 4 Cl at respective concentrations. Blue: DAPI; green: LC-3B and ATG-7; red: ATG-5 and Beclin-1. Scale bar: 5 μm. Images of multiple fields at 63× magnification were taken with oil immersion. c The number of LC-3B puncta relative to the cell area (10 cells per condition) was quantified using ImageJ. p < 0.0012. d At 2 h post-infection, NH 4 Cl was added at the indicated concentrations. Intracellular CFUs were demonstrated after 5 days of infection. p < 0.0195, p < 0.0042. n = 5 experiments. e Total protein was extracted from the above cells and western blotting was performed. A representative blot depicting the levels of p-AMPK, p-mTOR, p38 MAPK, LC-3 and p62/SQSTM1 in the control, ornithine or NH 4 Cl treated and Mtb H37Rv-infected macrophages is shown. Normalized fold intensities of p-AMPK, p < 0.0013, p < 0.0032, p < 0.0051; p-mTOR, p < 0.0017, p < 0.0027, p < 0.0018; p38 MAPK, ns not significant; and p62 levels p < 0.0191, p < 0.0072 in Mtb -infected and ornithine or NH 4 Cl treated macrophages compared with the levels in the uninfected control. n = 3 experiments. f At 2 h post-infection, ornithine and compound C were added at indicated concentrations. Intracellular CFUs were demonstrated after 5 days of infection. n = 5 experiments. Data are presented as the mean ± SD and analyzed using paired two-tailed t test. g Schematic representation of ornithine restricting Mtb growth in AMs. Red color indicates inhibitory line and green arrows indicates activation. Full size image Next, we examined the effect of ammonia on autophagy in Mtb -infected AMs and KCs. NH 4 Cl (25 mM) significantly inhibited the expression of LC-3B, ATG-5, ATG-7 and Beclin-1 in Mtb -infected AMs and KCs as demonstrated by confocal microscopy (Fig. 6b ). We also observed less LC-3B puncta formation in Mtb -infected AMs and KCs (Fig. 6c ) treated with NH 4 Cl compared to those treated with ornithine. The mean immunofluorescence intensities for LC-3B, ATG-5, ATG-7 and Beclin-1 were significantly higher in Mtb -infected AMs treated with ornithine than in Mtb- infected AMs treated with NH 4 Cl (Supplementary Fig. 11 ). Similarly, the mean immunofluorescence intensity of Mtb -infected KCs was significantly higher than Mtb -infected KCs treated with NH 4 Cl. Furthermore, treatment of Mtb -infected AMs and KCs with NH 4 Cl (5 and 25 mM) significantly enhanced Mtb growth in AMs and KCs in a concentration-dependent manner compared with the untreated controls (Fig. 6d ). Among the signaling pathways, 5′ adenosine monophosphate-activated protein kinase (AMPK), mitogen-activated protein kinases (MAPK) and mammalian target of rapamycin (mTOR) are the major factors that regulate autophagy [15] . The levels of phosphorylated AMPK were significantly upregulated while mTOR and p62 were downregulated in Mtb -infected KCs vs. uninfected KCs (Fig. 6e ). In contrast, Mtb infection did not enhance the phosphorylated AMPK level in AMs. Culturing of Mtb -infected AMs with ornithine upregulated p-AMPK to a level similar to that of Mtb -infected KCs (Fig. 6e ). We also found that culturing of Mtb -infected KCs with ammonia inhibited p-AMPK expression, but not MAPK expression. Similarly, culturing Mtb -infected KCs with nor-NOHA inhibited p-AMPK expression (Fig. 6e ). Additionally, the AMPK inhibitor compound C enhanced Mtb growth in KCs (Fig. 6f ) and downregulated the autophagy (Supplementary Fig. 12 ). In summary, our findings demonstrated that ornithine reduces ammonia levels, enhances AMPK phosphorylation, increases autophagy and inhibits Mtb growth in AMs and KCs (Fig. 6g and Supplementary Fig. 15 ). Imidazole inhibits Mtb growth by reducing cytochrome P450 To examine whether ornithine and imidazole have a direct effect on Mtb growth, we treated Mtb H37Rv broth cultures with ornithine and imidazole at 1, 5 and 10 mM daily and measured the OD 600 of 10 ml aliquots of Mtb H37Rv cultures (10 4 ) for a period of 5 days using spectrophotometer. Imidazole at 10 mM concentration significantly inhibited Mtb growth ( p < 0.0029 on the 4th day and p < 0.001 on the 5th day) in broth culture (Supplementary Fig. 13a ). In contrast, ornithine had no direct effect on Mtb growth. Mycobacterial cytochrome P450 monooxygenases (CYPs) are essential for Mtb growth, survival and virulence, thus possessing effective anti-mycobacterial activity [16] . Previous studies found compounds like azole inhibit CYPs. To investigate the effect of imidazole on Mtb CYPs, we treated Mtb H37Rv broth cultures with imidazole at 10 mM concentration daily for 4 days and evaluated mRNA expression of 20 CYP genes in treated cultures on days 3 and 4 by RT-PCR. We found that 18 of 20 CYPs were expressed in Mtb cultures (Supplementary Fig. 13b ). Among them, CYP51 , CYP130 , CYP128 and CYP121 were downregulated in Mtb treated cultures on day 4 compared with untreated Mtb culture, suggesting that imidazole inhibits expression of the CYPs described above to inhibit Mtb growth directly. Ornithine and imidazole restrict Mtb growth in the lungs We examined the effect of ornithine and imidazole on the lung bacterial burden in Mtb -infected mice. Mice were infected with Mtb H37Rv and treated with different concentrations of ornithine and imidazole (Fig. 7a ), followed by the evaluation of these metabolite levels in the lungs by LC-MS at four different time points (15 min and 2, 6, and 24 h) after intranasal delivery (Supplementary Fig. 14a ). After 15 min, both ornithine and imidazole concentrations were high in the lungs indicating that these metabolites were properly delivered. Ornithine was stable even at 24 h after the delivery whereas a very low amount of imidazole was observed (Supplementary Fig. 14b ). Fig. 7: Ornithine and imidazole restrict Mtb growth in the lungs. C57BL/6 mice were infected with 100 CFU of aerosolized Mtb H37Rv, and then treated with ornithine and imidazole at varying concentrations. a Schematic representation of Mtb infection and intranasal delivery of the compounds. b , c Bacterial burden in the lungs measured after one-month post-infection and post-treatment. Data are representative of three independent experiments ( n = 5 mice per group). Data are expressed as the mean ± SD. p < 0.0015. c Mtb- infected mice were treated in combination of ornithine/imidazole, one group treated with 1000/100 mg/kg, other as 2500/300 mg/kg and last group as 5000/600 mg/kg. p < 0.0029. d – f At one-month post - infection and post-treatment, the lungs of the uninfected control, Mtb- infected, ornithine or imidazole treated mice were isolated and formalin-fixed. Paraffin-embedded tissue sections were prepared, and hematoxylin and eosin staining was performed. Inflamed lung areas were compared among the groups. d A representative figure is shown. e Percentage of the lung lesions was calculated. p < 0.0024, p < 0.0192. f Paraffin-embedded lung tissue sections were analyzed by confocal microscopy to evaluate LC-3B (green), F4/80 (far-red) staining as well as their colocalization. Scale bar: 10 μm. A representative micrograph of LC-3B in lungs is shown. Images of multiple fields at 63× magnification were taken with oil immersion. g The immunofluorescence intensity (A.U.) of LC-3B are shown. Data are representative of three independent experiments. Five mice per group were used for each independent experiment. p < 0.0013. Statistical analysis was performed using paired two-tailed t test and data are represented as the mean ± SD. Full size image Ornithine treatment significantly reduced lung bacterial burden compared with PBS treatment in infected mice that were evaluated at 1-month post-infection (Fig. 7b ). A similar reduction in Mtb burden was observed in the lungs of imidazole treated mice compared with PBS treated mice (Fig. 7b ). Furthermore, the combination of both ornithine (5000 mg/kg) and imidazole (600 mg/kg) inhibited bacterial burden in the lungs more efficiently than when administered alone (Fig. 7c ). Histological analysis indicated that the number of lesions throughout the lungs was reduced significantly in ornithine and imidazole treated Mtb -infected mice compared with PBS treated Mtb -infected mice (Fig. 7d, e ). To demonstrate whether ornithine enhances autophagy in Mtb -infected lungs, we examined LC-3B expression in lung sections by confocal microscopy. Autophagy was increased in ornithine treated Mtb -infected lungs compared with PBS treated Mtb -infected lungs (Fig. 7f ). The mean immunofluorescence intensity of LC-3B was significantly higher in ornithine treated Mtb -infected lungs compared with PBS treated Mtb -infected lungs (Fig. 7g ). In contrast, imidazole treatment had no effect on autophagy in Mtb -infected lungs (Fig. 7f ). Macrophages are professional phagocytes that play an important role in controlling Mtb infection and disease progression [17] . The lungs are the target organs of Mtb infection in which AMs serve as the primary defense against Mtb [18] . AMs facilitate the establishment of Mtb at least during the initial stages of the infection and Mtb experiences less stress and maintains higher replication activity in AMs than in the other macrophage subtypes [19] , [20] . Therefore, Mtb appears to alter the function of AMs to facilitate its active growth in the lungs. In the case of extra-pulmonary sites, Mtb infection in the liver is very rare due to the restriction of the infection by KCs [21] . Despite the phagocytic nature of these two macrophage populations, Mtb replicates predominantly in the lungs but not in the liver. Previous studies have shown that in Mtb -infected mice, the liver has the lowest Mtb burden, consistent with more efficient clearance of bacteria with no recurrence [22] , [23] . In the current study, we found that KCs restricted Mtb growth more efficiently than AMs and PMs which is in line with the observations that demonstrated the role of KCs in bacterial clearance [24] . Monocytes are recruited at the site of infection to control TB growth [25] . We found Mtb growth in BDMs was similar to AMs and PMs but higher when compared to KCs. We chose BDMs for our studies because these cells infiltrate various tissues, are constitutively recruited during infection [26] and undergo differentiation to tissue-specific macrophages. Our results suggest that tissue-resident macrophages acquire their phenotype and functional capacity during their development from monocytes [27] . Furthermore, we also show that restriction of Mtb growth by KCs seems to be cytokine and TLR independent mechanism as AMs and KCs both produced an equivalent amount of cytokines and expressed similar levels of TLR’s. This could be attributable to the fact that macrophages use diverse mechanisms to kill Mtb . Macrophages display a high level of plasticity and the activation status of macrophages is critical for the development of host immune responses against invading pathogens [28] . It has been demonstrated that macrophages undergo different programs of activation, rendering them proinflammatory and microbicidal (M1), or immunosuppressive and tissue repairers (M2) [29] . Inducible nitric oxide synthase (iNOS) and type-I arginase (Arg-I) are widely used markers for the characterization of M1 and M2 phenotypes [30] . Here, we found similar expression of iNOS (M1) and Arg-1 (M2) in Mtb -infected AMs, PMs and KCs, suggesting that macrophage-polarized activation states are not involved in restricting Mtb growth. ROS and NO directly kill Mtb [31] and we found Mtb -infected AMs, PMs and KCs produced similar levels of ROS. In contrast, Mtb -infected KCs produced lower amounts of NO compared with those in other groups of infected macrophages. This may be because of the higher arginase activity of KCs, in which both iNOS and Arg-1 compete for the substrate L-arginine and the predominant enzyme (either iNOS or Arg-1) activated in macrophages in response to infection [32] and is likely associated with Mtb clearance [9] , [33] . During Mtb infection, the type of macrophage cell death is effective in controlling the infection and disease development [34] . Previous studies have shown that Mtb -infected macrophages trigger apoptosis, which is considered beneficial to the host [35] , and apoptotic cell death in Mtb -infected macrophages results in mycobacterial killing [36] . We found that Mtb -infected AMs, PMs and KCs were equally apoptotic, suggesting that efficient clearance of Mtb by KCs is not due to increased apoptosis and this led us to investigate alternate defense mechanisms in KCs. Autophagy acts as a first-line defense mechanism capable of eliminating intracellular bacteria, including Mtb [37] . Numerous studies have uncovered the role of autophagy against Mtb [38] , [39] which confers protection against TB by reducing bacterial burden and inflammation [40] . Similarly, our in vitro experiments revealed that Mtb -infected KCs had increased autophagic activity compared with Mtb -infected AMs and PMs, with autophagy induction being comparable to that induced by Rapamycin. However, AMs and PMs exhibited similar or lower levels of autophagy and failed to eliminate Mtb . Simultaneously, we also demonstrated that Mtb- infected AMs and PMs hampered the autophagic process by blocking maturation of autophagosomes, since p62 in these cells was not degraded. This may be attributable to the development by Mtb of the capacity to suppress host autophagy responses as a strategy to survive inside AMs, which is in accordance with previous studies [41] . Notably, Mtb causes nutritional imbalance which activates autophagy in infected macrophages. In this scenario, AMs, PMs and KCs should demonstrate similar autophagic activity but interestingly, we found KCs to be more autophagic. This provided evidence that alternate pathways are activated specifically in KCs that play a significant role in generating enhanced autophagy. Furthermore, inhibiting autophagy and molecules involved in regulating autophagy enhanced Mtb growth in KCs indicating enhanced autophagy in KCs contributes to the clearance of Mtb . Our findings suggest that specific pathways trigger autophagy in Mtb -infected liver cells. Cellular metabolism regulates autophagy; however, autophagy has a great impact on metabolic homeostasis of the liver [42] and some amino acids or their downstream metabolites, considered as antimicrobial agents [43] . Using a metabolomics approach, we identified 25 specific metabolites that were differentially generated in Mtb -infected AMs and KCs. Among these metabolites, ornithine and imidazole in Mtb -infected KCs and acetylcholine (Ach) in Mtb -infected AMs were classified as the best discriminators. Ornithine is a nonessential amino acid produced as an intermediate molecule in the urea cycle [44] . It is synthesized from L-arginine in the liver and involved in the regulation of several metabolic processes [45] . The metabolism of L-arginine and other metabolites (mostly ornithine) in the urea cycle serves to dispose excess nitrogen by converting ammonia to urea (Supplementary Fig. 11 ). During mycobacterial infections, L-arginine metabolism in activated myeloid cells is critical to the outcome of the infection; however, a direct effect of the metabolites derived from L-arginine on Mtb growth has not been studied [46] . We found that high levels of ornithine in KCs contributed to Mtb clearance, and treatment of infected AMs with ornithine restricted Mtb growth, suggesting a vital role for ornithine in Mtb growth restriction. Furthermore, we found that ornithine enhanced autophagy, which attenuated Mtb growth. Previously, KCs were shown to not express TACO (phagosome coat protein); consequently, Mtb is degraded by phago-lysosomal fusion resulting in efficient mycobacterial clearance [47] .Our results demonstrated that elevated levels of ornithine in Mtb -infected KCs enhanced autophagy, thus restricted Mtb growth. Both of these studies emphasize that the liver constitutes an efficient mycobacterial clearance site due to the presence of KCs. It remains to be observed whether ornithine downregulates TACO in Mtb -infected AMs. Ammonia is the major nitrogenous end product utilized by Mtb for metabolic activity [48] . In general, Mtb uses ammonia as a type of nitrogen source, required for its growth and survival [49] and inhibits phago-lysosomal fusion [50] . In light of these observations, we found increased production of ammonia in AMs compared with KCs, while its levels were reduced after treatment with ornithine indicated that ornithine plays a crucial role in the removal of excess ammonia. Accordingly, we anticipated that due to unavailability of nitrogen source, Mtb might not actively replicates thereby Mtb infection is controlled. Moreover, our results are consistent with previous studies that reported the dual effect of ammonia on autophagy where at elevated concentrations, it impairs autophagy [51] and at lower concentrations it strongly activates autophagy [52] . In addition, AMPK is a major energy-sensing serine/threonine kinase involved in metabolic homeostasis which is activated in response to nutrient stress [53] . Previous studies have shown that AMPK can sense nitrogen stress induced by depletion of either ammonia or amino acids and inhibits mTOR [54] . Nevertheless, the effects of nitrogen stress on AMPK in mammalian cells during Mtb infection remains unknown. We found that ornithine supplementation reduced ammonia levels and enhanced AMPK phosphorylation in AMs during Mtb infection. We also confirmed that the presence of higher levels of ammonia negatively regulated AMPK phosphorylation and inhibited autophagy in KCs (Fig. 6f ). Our results are consistent with recent studies that reported the key role of AMPK in Mtb growth restriction [55] associated with mTOR inhibition under stress related conditions. Thus, ornithine metabolizes ammonia which was elevated in Mtb -infected AMs leading to nitrogen stress, as ammonia is a type of nitrogen source required for Mtb survival, resulting in the activation of nutrient sensor p-AMPK triggering autophagy. Inhibition of p-AMPK activity in KCs using compound C enhanced Mtb growth. Previous studies used compound C to inhibit AMPK activity [56] , [57] , but it can inhibit other signaling pathways [58] . We were not able to confirm our findings using siRNA to AMPK due to technical issues but will be confirmed in future studies. Taken together, our findings demonstrate that ornithine suppresses ammonia assimilation and activates AMPK-mediated autophagy in AMs and KCs leading to effective Mtb growth restriction. The other metabolite highly expressed in infected KCs was imidazole, which is a nitrogen-containing heterocyclic ring present in purines, histamine, histidine, and nucleic acids [59] . Imidazole derivatives possess several biological activities such as antitumor, antiviral and antitubercular activities [60] . In accordance with previous reports, we found that treating infected AMs with imidazole inhibited Mtb growth. Unlike ornithine, imidazole inhibited Mtb growth by directly killing Mtb rather than enhancing autophagy. Although imidazole is a potent inhibitor of autophagy [61] , we did not observe any effect on autophagy in Mtb -infected AMs. Imidazole is an azole drug that inhibits cytochrome P450 involved in lipid and steroid metabolism [62] . Our current in vitro and in vivo findings are consistent with previous studies that imidazole restricts Mtb growth through inhibition of genes ( CYP51 , CYP130 , CYP128 and CYP121 ) involved in cytochrome P450. Thus, inhibition of these CYP s leads to impaired metabolic activity resulting in loss of nutrient uptake and ultimately leading to growth arrest. In addition, we also validated the effects of ornithine and imidazole by challenging mice with Mtb H37Rv and found that ornithine and imidazole inhibited Mtb growth in the lungs. Apart from the above-outlined metabolites, we also found that the Ach level was increased in Mtb -infected AMs compared with that in Mtb -infected KCs. Mtb growth was attenuated in AMs treated with an Ach antagonist (atropine), suggesting that Ach blockade might be working through boosting antimicrobial defense mechanism of AMs. It is well known that Ach is a neurotransmitter that is a component of the nonneuronal cholinergic system, functions as a cross communication between microbes and immune system [63] and Ach receptors can suppress macrophage activity [64] . Our results suggest specific Ach receptor agonists/antagonists can be used to restrict Mtb growth in AMs. Moreover, a recent study reported that activation of gamma-amino butyric acid (GABA), a principal inhibitory neurotransmitter, enhanced antimicrobial responses through autophagy against intracellular bacterial infection [65] . This suggests that Ach production in AMs may inhibit antimicrobial responses by suppressing autophagy against Mtb . Thus, better understanding of the functional relevance of these neurotransmitters regarding the host defense system would probably be useful for the development of therapeutic strategies against Mtb . Our study further demonstrated that AMs possess specific metabolic pathways to inhibit Mtb growth, but the impact of Ach signaling on the host immune defense system against Mtb remains to be explored. In conclusion, our study demonstrated that KCs restrict Mtb growth more effectively than AMs due to the production of ornithine and imidazole. Furthermore, understanding the immune-metabolic mechanisms may reveal attractive targets for the control of TB and enable identification of complementary drug targets to limit TB infection. Mice All mouse experiments were performed with specific pathogen-free female C57BL/6 mice that were typically 6–8 weeks old, purchased from the Jackson Laboratory. These animals were housed in the animal care facility and received human care in accordance with the National Institutes of Health guidelines for animal research. Ethics statement All the animal studies were approved by the Institutional Animal Care and Use Committee of the University of Texas Health Science Center at Tyler (Protocol #605). The animal procedures involving the care and use of mice were undertaken in accordance with the guidelines of the NIH/OLAW (Office of Laboratory Animal Welfare). Reagents L-ornithine monohydrochloride was purchased from Kyowa Hakko Bio (150002; Tokyo, Japan). Imidazole (15513), atropine (A0132), rapamycin (R8781), Bafilomycin A1 (SML1661), 5-Aminoimidazole-4-carboxamide-1-β-D-ribo furanoside (AICAR; A9978, compound C (171260) and ammonium chloride (NH 4 Cl; A9434) were obtained from Sigma-Aldrich. Nor-omega-hydroxide-L-arginine (nor-NOHA; 10006861) was purchased from Cayman chemicals and recombinant IL-4 (carrier-free) from eBioscience (574304). γ irradiated Mtb H37Rv (γ- Mtb ) was obtained from BEI Resources. Isolation of mouse alveolar macrophages Mouse AMs were isolated from the control mice by bronchoalveolar lavage. Briefly, mice were euthanized by CO 2 asphyxiation. The trachea was then cannulated following a midline neck incision, and the lungs were lavaged five times with 2 ml of ice-cold PBS. We pooled AMs from three mice for each experiment. Alveolar cells were isolated from the lavage fluid by centrifugation at 1600 RPM for 10 min, and cells were plated in a 12-well tissue culture plates at a density of 3 × 10 6 /well. The cells were incubated for 24 h at 37 °C with 5% CO 2 to allow the alveolar macrophages to adhere onto the plates. Subsequently, the non-adherent cells were removed by washing three times with normal PBS. Adherent cells were resuspended in RPMI-1640. Approximately 95% of the cells expressed both F4/80 and CD11c, as demonstrated by flow cytometry (Supplementary Fig. 1a ). Isolation of mouse peritoneal macrophages Mice were euthanized by CO 2 asphyxiation followed by cervical dislocation. Subsequently, a small incision was made along the bottom midline of the peritoneum, and the abdominal skin was retracted to expose the transparent peritoneal skin. Peritoneal cells were collected by injecting 5 ml of ice-cold PBS into the peritoneal cavity thrice. We pooled PMs from three mice for each experiment. The cells were then separated by centrifugation at 1600 RPM for 10 min, and cells were plated in a 12-well tissue culture plates at a density of 3 × 10 6 /well and incubated for 24 h at 37 °C with 5% CO 2 to allow adherence of macrophages onto the plates by removal of the non-adherent cells by washing three times with normal PBS. Adherent cells were resuspended in RPMI-1640 and were further incubated for 3 days for the respective experiments. Around 94% of the cells expressed F4/80, as demonstrated by flow cytometry (Supplementary Fig. 1b ). Isolation of mouse Kupffer cells Mice were euthanized by CO 2 asphyxiation, and then their livers were perfused. Briefly, the peritoneal cavity was cut open, and an incision was made on the portal vein to drain the blood followed by perfusion with ice-cold PBS through the inferior vena cava until the liver turned pale yellow. The liver was harvested from the control mice and placed into 30-mm dishes containing 2 ml of Hank’s balanced salt solution (HBSS). We pooled KCs from three mice for each experiment. The tissues were minced with scissors into pieces no larger than 2–3 mm, and the fluid was discharged onto a 70-μm filter (BD Biosciences, San Jose, CA) that had been pre-wetted with 1 ml of PBS containing 0.5% bovine serum albumin (BSA, Sigma-Aldrich) over a 50-ml conical tube. The syringe plunger was then gently used to disrupt the liver tissue before washing the filter with 2 ml of cold PBS. Liver cells were separated by centrifugation at 1600 RPM for 10 min. The pellet was resuspended in a 35% Percoll gradient (20 ml) and then layered on a 67% Percoll gradient (13 ml) followed by centrifugation at 600 × g for 20 min. Nonparenchymal cells (KCs) from the interface between the two density cushions of 35% with 67% Percoll were then resuspended in PBS followed by centrifugation at 1600 RPM for 10 min. The total number of viable cells was examined with the trypan blue exclusion method. KCs were plated in to a 12-well tissue culture plates at a density of 3 × 10 6 /well, incubated for 24 h at 37 °C with 5% CO 2 to permit adherence of KCs and subsequent removal of non-adherent cells by washing three times with normal PBS. The adherent cells were finally resuspended in RPMI-1640. Approximately 90% of the cells expressed both F4/80 and CD68 as demonstrated by flow cytometry (Supplementary Fig. 1c ). Isolation of BMDMs Mice were euthanized by CO 2 asphyxiation followed by cervical dislocation. To generate bone marrow cells, femurs and tibias were harvested and were dipped in ethanol and followed by PBS. The ends of the bones were cut off with sharp scissors and the bone marrow flushed out with ice-cold PBS using a syringe and 25G needle (approximately 3 ml per fibula and 2 ml per tibia) and dispersed the aggregates by passing cell suspension through 70-µM filter. Cells were centrifuged at 300 × g for 6 min and then resuspended cell pellet with 1 ml RBC lysis for 5 min at room temperature and neutralized the lysis buffer by adding PBS followed by centrifugation at 300 × g for 6 min and then cells were resuspended in RPMI-1640. Monocytes were enriched from bone marrow cells by using Easy step mouse monocyte isolation kit (STEM CELL Technologies) according to manufacturer’s protocol. The eluted fraction was stained for CD11b and Ly6C, and ~94% of pure monocytes were obtained as demonstrated by flow cytometry (Supplementary Fig. 1d ). Next, monocytes were plated in to a 12-well tissue culture plates at a density of 3 × 10 6 /well, incubated for 24 h at 37 °C with 5% CO 2 to allow adherence of the cells onto the plates followed by removal of the non-adherent cells by washing three times with normal PBS. The adherent cells were resuspended in RPMI-1640. Mtb infection of macrophages and colony-forming unit assays AMs, PMs, KCs and BDMs were infected with Mtb H37Rv at an MOI of 1:2.5 (1 monocyte/macrophage and 2.5 Mtb ). This MOI was based on the viability of macrophages at different MOIs for up to 7 days p.i. More than 90% of the macrophages were viable at this MOI. Cells were incubated for 2 h at 37 °C in a humidified 5% CO 2 atmosphere, washed to remove extracellular bacilli and cultured in RPMI-1640 containing 10% heat-inactivated fetal bovine serum. To quantify the intracellular growth of Mtb H37Rv, infected macrophages were cultured for 5 days, after which the supernatant was aspirated, and the macrophages were lysed. Bacterial suspensions in cell lysates were ultrasonically dispersed, serially diluted and plated in triplicate on 7H10 agar, and the colonies were counted after 21 days. Cell treatment AMs, PMs and KCs were infected with Mtb H37Rv at an MOI of 1:2.5 (1 macrophage and 2.5 Mtb ). Cells were incubated for 2 h at 37 °C in a humidified 5% CO 2 atmosphere, washed to remove extracellular bacilli and cultured in RPMI-1640 containing 10% heat-inactivated fetal bovine serum followed by the addition of ornithine, imidazole and atropine (Sigma-Aldrich) at concentrations of 1, 5 and 10 mM. After 72 h, AMs, PMs and KCs were harvested for further experiments. Cytokine ELISAs AMs, PMs and KCs were infected with Mtb H37Rv, and culture supernatants were collected after 72 h and stored at −70 °C until concentrations of TNF-α, IL-6, IL-1β and IL-10 (eBioscience) were measured by ELISA according to the manufacturer’s protocol. Measurement of ROS production To evaluate the intracellular ROS levels, AMs, PMs and KCs were seeded in 24-well tissue culture plates at a density of 1 × 10 6 /well and infected with or without Mtb H37Rv. After 24 h of infection, the cells were harvested and replenished with 100 μl RPMI-1640 and incubated in the presence of 20 μM 2′, 7′-dichlorofluorescein diacetate (DCFDA) at 37 °C and 5% CO 2 for 15 min by using DCFDA Cellular ROS detection assay kit (Abcam, ab 113851). As a positive control, the cells were treated with 55 mM Tert-Butyl Hydrogen Peroxide (TBHP) for 4 h. The fluorescence intensity, reflecting the intracellular ROS levels, was immediately measured using a FACS Calibur flow cytometer (BD Biosciences, San Jose, CA). The ROS levels are expressed as a histogram of mean fluorescence intensities generated from 10,000 cells. Nitric oxide detection AMs, PMs and KCs were cultured in 24-well tissue culture plates at a density of 1 × 10 6 /well, and were infected with or without Mtb H37Rv, and culture supernatants were collected after 72 h. The NO levels of the supernatants were indirectly quantified by measuring the concentration of its products nitrate and nitrite in the supernatants. The NO measurement was performed with the nitrate and nitrite colorimetric assay kit (Cayman Chemicals) according to manufacturer’s protocol immediately after collecting the supernatants. Briefly, 80 µl of the culture supernatant was incubated with 10 µl of each enzyme cofactor and nitrate reductase mixture for 1 h at room temperature followed by addition of 50 µl of each Griess reagent R1 and R2. Formation of azo compound was monitored at optical density of 540 nm after 10 min of incubation using Versa max microplate reader (Molecular Devices). Arginase activity Arginase activity was evaluated in protein extracts by measuring the conversion of L-arginine into L-ornithine with the arginase activity assay kit (Bio Vision) according to the manufacturer’s instructions. Briefly, AMs, PMs and KCs were cultured at 1.5 × 10 6 /well in 24-well tissue culture plates and infected with or without Mtb H37Rv and some of them were treated with IL-4 (10 ng/ml) and nor-NOHA (10 µM). After 72 h of infection and treatment, the cells were washed with PBS and homogenized on ice with ice-cold arginase assay buffer containing the protease inhibitor (provided in the kit) followed by centrifugation at 10,000 × g for 5 min at 4 °C. The lysates (40 µl) were transferred in to a 96-well microplate in duplicates and incubated with 10 µl of the substrate mix for 20 min at 37 °C. Subsequently, the samples and standards were mixed with 50 µl of the reaction mixture containing 42 μl arginase assay buffer, 2 μl enzyme mix, 2 μl developer, 2 μl converter enzyme and 2 μl oxi red probe and optical density of the samples was measured at 570 nm using Versa max microplate reader (Molecular Devices). Assessment of intracellular ammonia AMs and KCs were seeded at 2 × 10 6 /well in a 24-well tissue culture plates and infected with or without Mtb H37Rv for 72 h. Cells were washed with PBS and lysed in ammonia assay buffer provided in the ammonia assay kit (Abcam, ab83360, Cambridge, UK) and measured intracellular NH 4 + /NH 3 levels by following the manufacturer’s instructions. Briefly, samples were set up using 25 μl of cell lysates added to 25 μl of assay buffer in duplicate in a 96-well microplate. The reaction mixture was prepared as a master mix with each reaction consisting of 42 μl ammonia assay buffer, 2 μl oxi red probe, 2 μl Enzyme Mix, 2 μl developer, and 2 μl of the converting enzyme. This reaction mixture (50 μl) was added into the samples and standard wells, which were then mixed and incubated for 1 h at 37 °C in the dark. Optical density was measured at 570 nm using a Versa max microplate reader (Molecular devices). Measurement of apoptosis by phosphatidyl serine exposure assay A quantitative assessment of apoptosis was performed using a fluorescein isothiocyanate (FITC) Annexin-V Apoptosis Detection Kit I (BD Biosciences, Waltham, MA). Briefly, macrophages were infected with Mtb H37Rv at an MOI of 1:2.5 (1 macrophage and 2.5 Mtb ). After 72 h, macrophages were harvested, washed once in PBS and then once in binding buffer and resuspended in binding buffer (1 × 10 6 cells/ml). After 100 µl of cells was transferred to a tube, 5 µl of FITC-conjugated Annexin-V was added, followed by incubation for 15 min in the dark. Later 5 µl of propidium iodide (PI) was added and immediately analyzed by the FACS Calibur flow cytometer (BD Biosciences, San Jose, CA). Data from 10,000 cells were collected in each data file. Four different populations of cells are easily distinguished: those that were unlabeled (viable cells), those that had bound Annexin V-FITC only (early apoptotic), those that had been stained with PI (necrotic) and those that both labeled with both Annexin V-FITC and PI (late apoptotic/necrotic cells). The fluorescence distribution was displayed as a two-color dot plot analysis and the percentage (%) of fluorescent cells in each quadrant was demonstrated. Measurement of apoptosis by Apo-Direct TUNEL assay Apoptosis was confirmed by the determination of single DNA strand breaks by use of the TUNEL assay (BD Biosciences Waltham, MA). In brief, macrophages were infected with Mtb H37Rv at an MOI of 1:2.5 (1 macrophage and 2.5 Mtb ). After 72 h, macrophages were harvested using PBS-EDTA, washed twice in PBS and fixed in 1% paraformaldehyde and 70% cold ethanol in PBS. After overnight incubation at −20 °C, cells were washed in washing buffer, resuspended in 50 μl of DNA labeling solution (provided in the kit) and incubated at 37 °C. After 60 min, the cells were washed twice in rinsing buffer, and 500 μl of propidium iodide/RNase A solution was added and incubated in the dark. After 30 min, the cells were analyzed by FACS. Assessment of autophagic activity by flow cytometry Mtb induced autophagy was detected using a LC-3 antibody-based assay kit (Millipore’s FlowCellect) according to the manufacturer’s instructions. In brief, macrophages were infected with Mtb H37Rv at an MOI of 1:2.5 (1 macrophage and 2.5 Mtb ). After 72 h, macrophages were harvested using PBS-EDTA, washed once in 1X assay buffer (provided in the kit) followed by centrifugation at 300 × g for 5 min. The pellet was resuspended in 1X autophagy reagent B and immediately centrifuged at 300 × g for 5 min. The supernatant was aspirated, and the pellet was again resuspended in 95 µl of 1X assay buffer + 5 µl of 20X anti-LC-3/Alexa Fluor® antibody for 30 min at room temperature in the dark. The cells were washed once with 1X assay buffer to remove unbound antibody followed by centrifugation at 300 × g for 5 min and then resuspended in 1X assay buffer and then the data was acquired by FACS. Western blot To detect the expression of key autophagy-relevant proteins, AMs, PMs and KCs were cultured (3 × 10 6 cells/well in 12-well plates) with or without Mtb . After 72 h of infection, AMs, PMs and KCs were lysed in the lysis buffer (M-PER protein extraction reagent with a protease inhibitor cocktail; Thermo Scientific) and the total protein amount in these lysates was evaluated using a BCA protein assay kit (Thermo Scientific) according to the manufacturer’s protocol. Approximately 25 µg of protein was resolved by 10% SDS-PAGE alongside a precision plus protein standard marker (Bio-Rad). Resolved proteins were transferred onto PVDF membranes followed by blocking with 5% skimmed milk for 1 h at room temperature. They were then probed overnight at 4 °C for LC-3A/B (cell signaling,12741, 1:1000) LC-3B (cell signaling, 3868, 1:1000), p62/SQSTM1 (cell signaling, 8025,1:1000), ATG-5 (Abcam, 108327, 1:1000), ATG-7 (Abcam, 133528, 1:10000) Beclin-1 (Abcam, 62557, 1 µg/ml), p-mTOR (cell signaling, 5536, 1:1000), p-AMPKA (cell signaling, 50081,1:1000), p38 MAPK (cell signaling, 8690,1:1000) and GAPDH (Cell Signaling, 8884, 1:1000) in 5% skimmed milk. Membranes were washed and incubated with an anti-rabbit IgG HRP-linked secondary antibody (cell signaling, 7074P2, 1: 3,000/5,000). Protein bands were detected using the Super-Signal™ west Pico Plus chemi luminescent substrate (Thermo Scientifics, 34577). Images were acquired in parallel from a single gel. Respective band densities were quantified using the ImageJ software (NIH, USA). RNA extraction and quantitative real-time PCR Mouse AMs, PMs and KCs were cultured in the presence or absence of Mtb H37Rv for 72 h, after which total RNA was isolated using TRIzol (Invitrogen) according to the manufacturer’s instructions. Complementary DNA (cDNA) was generated from 0.5 mg of RNA and random hexamer primers using a Maxima First Strand cDNA Synthesis Kit for RT-qPCR (BIO-RAD) according to the manufacturer’s instructions and real-time PCR was performed. Gene expression levels of LC-3B, ATG-5, ATG-7 and Beclin-1 were evaluated using SYBR Green Master Mix (Qiagen), gene-specific primers (Sigma-Aldrich) and an ABI Prism 7600. The mouse primer sequences used for PCR were as follows: LC-3B, 5″-ATGCCGTCCGAGAAGACCTTC-3″ (forward) and 5″-TTACACAGCCATTGCTGTC-3″ (reverse); ATG-5, 5″-TGCTGAAGGCTGTAG GAGAC-3″ (forward) and 5″-CGAGGCCACCAGTTTAAGGA-3″ (reverse); ATG-7, 5″-GTTGAGCGGCGACAGCATTAG-3″ (forward) and 5″-GGCACTATTAAAGGGGGCGA-3″ (reverse); Beclin-1, 5″-CAG GAACTCACAGCTCCATTACT-3″ (forward) and 5″-TAGCCTCTTCCTCCTGGGTC-3″ (reverse); iNOS, 5″-TCCTCACTGGGACAGCACAGA-3″ (forward) and 5″-GTGTCATGCAAAATCTCTCC ACTGCC-3″ (reverse); Arg-1, 5″-GGAATCTGC ATGGGCAACCTGTGT-3″ (forward) and 5″-AGGGT CTACGTCTCGCAAGCC-3″ (reverse); GAPDH, 5″-GCCATCAATGACCCCTTCATT-3″ (forward) and 5″-TTGACGGTGCCATGGAAT TT-3″ (reverse). All gene expression levels were normalized to GAPDH internal controls, and the fold changes were calculated using the 2 −ΔΔCT method. Total RNA extraction from Mtb H37Rv and quantitative PCR Mtb H37Rv were cultured in 10 ml Middlebrook 7H9 broth (BD, Franklin Lakes, NJ, USA) supplemented with 10% oleic acid, albumin, dextrose, catalase enrichment (BD), and 0.5% (v/v) glycerol in a 37 °C incubator for 2–3 weeks. An aliquot (7 ml) of the culture was then transferred into 15 ml screw-cap tubes and centrifuged at 2200 × g for 10 min at 4 °C. The pellet containing the mycobacterial cells was washed with 2 ml Tris-EDTA buffer (pH 7.5) to remove the excess 7H9 broth by tapping the tube, and then centrifuged again. The pellet was resuspended in 1 ml TRIzol reagent (Invitrogen) and mechanically disrupted using sonicator for 10 s twice and then RNA was extracted according to the manufacturer’s instructions. To eliminate genomic DNA contamination, DNA was digested using a TURBO DNA-free Kit (Ambion, Life Technologies, Carlsbad, CA, USA). Complementary DNA (cDNA) was generated from 0.5 mg of RNA by using random hexamer primers and a Maxima First Strand cDNA Synthesis Kit for RT-qPCR (BIO-RAD) according to the manufacturer’s instructions and real-time PCR was performed. Gene expression levels of 20 Mtb cytochrome P450’s were demonstrated using SYBR Green Master Mix (Qiagen), gene-specific primers (Sigma-Aldrich) and a Quant studio 7 flex (Applied Biosystems) in duplicates. 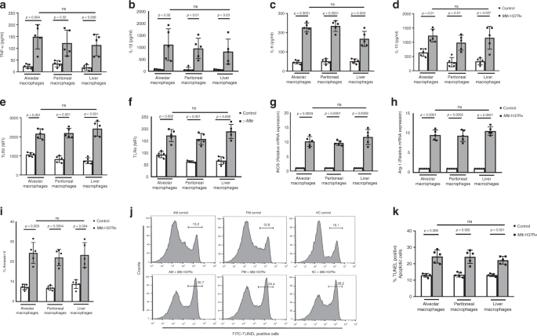Fig. 2:Mtbinduces equal cytokine levels and apoptosis in KCs, AMs and PMs. AMs, PMs and KCs from C57BL/6 mice were isolated and infected withMtbH37Rv as mentioned in Fig.1, and after 72 h, the (a) TNF-α.p< 0.0048 (b) IL-1β. p < 0.0241,p< 0.014 (c) IL-6 and (d) IL-10 cytokines levels in culture supernatants were measured by ELISA.p< 0.0144,p< 0.0129,p< 0.0077; ns not significant (e,f) AMs, PMs and KCs were also cultured with gamma-irradiatedMtb(γ-Mtb) for 24 h.eTLR-2.p< 0.0011,p< 0.0011 andfTLR-4 expression was demonstrated by flow cytometry.p< 0.0011. AMs, PMs, and KCs were infected withMtbH37Rv and after 72 h,giNOS andhArg-1 mRNA expression was demonstrated by real-time PCR. The mean ± SD of the fold change in mRNA levels in infected macrophages compared to uninfected macrophages is represented. AMs, PMs and KCs from C57BL/6 mice were isolated and infected withMtbH37Rv at an MOI of 1:2.5. After 72 h, apoptosis was demonstrated by the Phosphatidyl-serine exposure assay/Annexin-V/PI staining and confirmed by the TUNEL assay.iThe percentage of the early phase apoptotic cells is shown.p< 0.0031,p< 0.0041.jA representative flow cytometry plot for the TUNEL assay.kThe percentage of the late phase apoptotic cells is shown.p< 0.0033,p< 0.0013, ns: not significant. Statistical analysis was performed with paired two-tailed t test and presented as mean ± SD. Data represent the average of five independent experiments. The Mtb cytochrome P450 primer sequences used were listed in Supplementary Table 2 . All the gene expression levels were normalized to 16S rRNA as the internal control and the relative expression levels were evaluated. Immunofluorescence detection of autophagy-relevant proteins Confocal microscopy was performed to evaluate LC-3B, ATG-5, ATG-7 and Beclin-1 expression in AMs, PMs and KCs cultured with or without Mtb infection. These macrophages (3 × 10 6 /well) were plated in 12-well plates in 1 ml of antibiotic-free RPMI-1640 containing 10% heat-inactivated fetal bovine serum and incubated at 37 °C in a humidified 5% CO 2 atmosphere. Adherent cells were infected with Mtb H37Rv at an MOI of 1:2.5 (1 macrophage and 2.5 Mtb ). After 2 h, cells were washed to remove extracellular bacilli and cultured in RPMI-1640 containing 10% heat-inactivated fetal bovine serum for 72 h. Where indicated, ornithine, imidazole and NH 4 Cl were added to the cells after 2 h of infection and then the cells were incubated for 72 h. For immunostaining, cells were first briefly washed with PBS and then fixed with 4% paraformaldehyde for 15 min at room temperature and washed with PBST three times for 5 min each. Fixed cells were then incubated with 0.025% Triton X-100 in PBST for 10 min and subjected to three subsequent washes with PBST. Nonspecific binding was blocked by incubating the samples in 5% bovine serum albumin (BSA) in PBST for 1 h. The samples were then washed with PBST twice for 5 min each. Next, the samples were incubated in PBST overnight at 4 °C with the following dilutions of the primary antibodies; LC-3B (1:250), ATG-5 (1:250), ATG-7 (1:250), Beclin-1(1:250). Subsequently, the samples were thoroughly washed with PBST three times for 5 min each. Next, the cells were stained with the respective secondary antibodies at 1:500 dilutions (v/v) and washed again with PBST three times for 5 min each before mounting with the fluoroshield mounting medium containing DAPI. The mounted slides were then examined and analyzed under a laser-scanning confocal microscope (Zeiss LSM 510 Meta laser-scanning confocal microscope). Zen 2009 software (Carl Zeiss) was used for image acquisition. The images were then uniformly processed and quantified in each experiment using ImageJ NIH software. Representative images are shown from five independent experiments. Measurement of autophagic flux Formation of autophagosomes and autophagolysosomes in AMs, PMs and KCs cultured with or without Mtb infection was measured by using Premo TM Autophagy Tandem Sensor RFP-GFP-LC3B kit (Thermo Fischer Scientifics) according to the manufacturer’s instructions. AMs, PMs and KCs (3 × 10 6 /well) were plated in 12-well plates in 1 ml of antibiotic-free RPMI-1640 containing 10% heat-inactivated fetal bovine serum and incubated at 37 °C in a humidified 5% CO 2 atmosphere. Adherent cells were labeled with the autophagy sensor for 48 h and then infected with Mtb H37Rv at an MOI of 1:2.5 (1 macrophage and 2.5 Mtb ). After 2 h, cells were washed to remove extracellular bacilli and cultured in RPMI-1640 containing 10% heat-inactivated fetal bovine serum for 72 h. Where indicated, ornithine and imidazole were added to the cells after 2 h of infection and then the cells were incubated for 72 h. Some of the cells were also treated with chloroquine (50 µM) for 5 h before the cells were fixed and then mounted with fluoroshield mounting medium. The mounted slides were then examined and analyzed under a laser-scanning confocal microscope (Zeiss LSM 510 Meta laser-scanning confocal microscope). Zen 2009 software (Carl Zeiss) was used for image acquisition. The images were then uniformly processed and quantified in each experiment using ImageJ NIH software. Representative images are shown from three independent experiments. Small interfering RNA Freshly isolated AMs, PMs and KCs were transfected with small interfering RNAs (siRNAs) targeting LC-3B, ATG-5, ATG-7 and Beclin-1 or with control siRNA using transfection reagents (all from Santa Cruz Biotechnology). The efficiency of siRNA knockdown was measured by western blot shown in Supplementary Fig. 4 . In brief, 3 × 10 6 AMs/PMs or KCs were resuspended in 500 µl of transfection medium and transfected with siRNA (6 pmol). After 6 h, an additional 500 µl of 2X RPMI-1640 complete medium was added, and cells were cultured overnight into a 12-well plate. The next day, macrophages were washed and infected with Mtb H37Rv as outlined above, and CFU counts were demonstrated after 5 days. Aerosol infection of the mice with Mtb H37Rv Wild-type C57BL/6 mice were infected with Mtb H37Rv using an aerosol exposure chamber. In brief, Mtb H37Rv was grown to the mid-log phase in the liquid medium and then kept in aliquots at −70 °C. Bacterial counts were demonstrated by plating onto 7H10 agar plates supplemented with oleic albumin dextrose catalase (OADC). For infection, the bacterial stocks were diluted in 10 ml of normal saline (to 0.5 × 10 6 CFU/ml, 1 × 10 6 CFU/ml, 2 × 10 6 CFU/ml, and 4 × 10 6 CFU/ml) and placed in a nebulizer within an aerosol exposure chamber custom made by the University of Wisconsin. In the preliminary studies, groups of three mice were exposed to the aerosol at each concentration for 15 min. After 24 h, the mice were euthanized, and homogenized lung samples were plated onto 7H10 agar plates supplemented with OADC. The CFUs were counted after 14–22 days of incubation at 37 °C. The aerosol concentration that resulted in ~100 bacteria in the lungs was used for the subsequent studies. Ornithine and imidazole intranasal administration Mice were infected with ~100 CFU of Mtb H37Rv in an aerosol exposure chamber as outlined above. Next day, the infected mice were intranasally treated with ornithine (L-ornithine monohydrochloride; KYOWA HAKKO BIO Co., Ltd.) and imidazole (Sigma-Aldrich) at varying concentrations. In brief, mice were deeply anesthetized with ketamine plus xylazine (75 and 10 mg/kg i.p. injections) followed by intranasal administration of L-ornithine monohydrochloride (1000 mg/kg, 2500 mg/kg, or 5000 mg/kg) and imidazole (100 mg/kg, 300 mg/kg, or 600 mg/kg) twice a week for 30 days, while the control mice were injected with PBS (pharmaceutical grade; VWR life science). The highest dose was selected based on the LD50 provided in the manufacturer’s safety data sheet. After 30 days of treatment, the lungs were harvested to examine the CFU counts. In brief, the lungs were placed into 30-mm dishes containing 2 ml of 7H9 media and minced with scissors into pieces no larger than 2–3 mm. The fluid was discharged through a 70-μm filter (BD Biosciences, San Jose, CA) suspended over a 50-ml conical tube. The syringe plunger was then used to gently disrupt the lung tissue and the supernatant containing the cells was incubated for 2 h at room temperature. Finally, CFU assay was performed as outlined above. All the experiments were performed thrice with five mice in each group. Metabolome extraction and LC-MS AMs, PMs, KCs and BDMs (2 × 10 6 ) were cultured uninfected or infected with Mtb H37Rv as previously described. After 72 h of infection, BDMs and macrophages were washed twice with 5 ml of ice-cold normal saline solution. The cells were resuspended in 1 ml of methanol (80% v/v) on dry ice, then subjected to three freeze-thaw cycles between liquid nitrogen and 37 °C. After the third thawing, the samples were vortexed for 1 min followed by centrifugation at 20,160 × g for 15 min at 4 °C. Later, the supernatant containing the pellet was dried by a speedVac using no heat and stored at −80 °C. The metabolite pellet was shipped to the Children’s Medical Center Research Institute at UT Southwestern (Dallas, TX) for liquid chromatography-mass spectrometry (LC-MS). In brief, LC-MS was performed in the MRM mode on a triple quadrupole mass spectrometer with two different dilutions of sample plus four retention times and three quality control standards. To evaluate the delivery of ornithine and imidazole after intranasal administration, mice were infected, treated and their lungs were collected at four different time points (15 min, 2 h, 6 h and 24 h) after delivery as outlined above to extract the metabolome for LC-MS. In brief, 50 mg of lung tissue was homogenized with 300 μl of acetonitrile/water 80:20 (vol/vol) and subjected to three freeze-thaw cycles between liquid nitrogen and 37 °C. Next, they were rigorously vortexed for 1 min and then centrifuged at 20,160 × g for 15 min at 4 °C twice. The metabolite containing supernatant for quantification was shipped to the Children’s Medical Center Research Institute at UT Southwestern (Dallas, TX) for liquid chromatography-mass spectrometry (LC-MS). Immunohistochemistry After one-month of Mtb infection as well as treatment, mice were euthanized, and the lungs were inflated and fixed in 10% neutral buffered formalin (Statlab, McKinney, TX, USA) for 48 h to inactivate the infectious agent. Paraffin-embedded blocks were cut into 5 μm thick sections. For morphometric lesion analyses, the lung sections were stained with hematoxylin and eosin (H&E) and examined in a blinded manner to assess the lung lesions [66] . Briefly, the lesion area and percentage of each lung occupied by lesions was quantified for each lobe by using digital software (NIH ImageJ; developed at the U.S. National Institutes of Health and available on the Internet at https://imagej.nih.gov/ij/ ). Immunofluorescence staining of thin paraffin-fixed lung sections was also performed using confocal microscopy. Unstained sections of formalin-fixed lung tissue from paraffin blocks were first deparaffinized and rehydrated, followed by heat-induced antigen retrieval in citrate buffer (pH 6.0). Then, the lung tissue sections were incubated in 0.025% Triton X-100 in PBST for 10 min and washed 3 × 5 min using PBS. 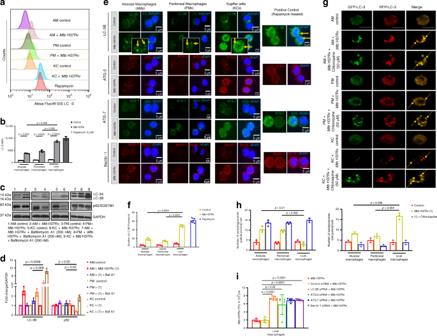Fig. 3: Kupffer cell autophagy is increased byMtbinfection. AMs, PMs, and KCs from C57BL/6 mice were infected withMtbH37Rv. After 72 h, LC-3 positive cells were evaluated by flow cytometry.aRepresentative flow cytometry plot for LC-3.bMean fluorescence intensity (MFI) of LC-3 expression.n= 3 experiments.p< 0.0024,p< 0.0064,p< 0.0051,p< 0.0058.cTotal protein was extracted from the above cells and western blotting was performed. A representative blot depicting the levels of LC-3 and p62/SQSTM1 in the control,MtbH37Rv-infected and bafilomycin A1 treated macrophages is shown. GAPDH was used as a loading control.dNormalized fold intensities of LC-3B, p62 levels inMtbH37Rv-infected macrophages relative to the levels in the uninfected control.n= 3 experiments.p< 0.0098,p< 0.0263,p< 0.028.eA representative micrograph of LC3-B, ATG-7, ATG-5 and Beclin-1 in AMs and KCs. Blue: DAPI; green: LC-3B and ATG-7; red: ATG-5 and Beclin-1. Images of multiple fields were taken at 63× magnification with oil immersion.fThe number of LC-3B puncta relative to the cell area was measured using ImageJ and quantified in 10 cells per condition.gMacrophages were labeled with an autophagy sensor expressing RFP-GFP-LC3B for 48 h. The labeled macrophages were then infected withMtbH37Rv for 72 h. The cells were fixed, and LC-3B was analyzed by confocal microscopy. Autophagosomes show both GFP (green) and RFP (red) signals. Autophagosome-lysosome fusion results in RFP-positive and GFP-negative dots. Scale bars: 5 µm.hQuantification of the number of LC-3B positive autophagosomes (yellow fluorescence) and autolysosomes (red fluorescence) in control,Mtb-infected macrophages followed by treatment with or without chloroquine is shown.n= 3 experiments.p< 0.0142,p< 0.0025,p< 0.0063,p< 0.0047.iKCs from C57BL/6 mice were isolated and transfected with siRNAs targeting LC-3B, ATG-5, ATG-7 and Beclin-1 or with control siRNA and then infected withMtbH37Rv. After 5 days, CFUs were counted.n= 5 experiments. Data are presented as the mean ± SD using paired two-tailed t test. Nonspecific binding was blocked with 5% BSA in PBST for 1 h, and the slides were washed 2 × 5 min with PBS. The slides were then incubated at 4 °C overnight in PBST with the appropriate dilutions of the following antibodies; anti-F4/80 (1:50), anti-LC-3B, anti-ATG-5, anti-ATG-7 and anti-Beclin-1 (1:100). 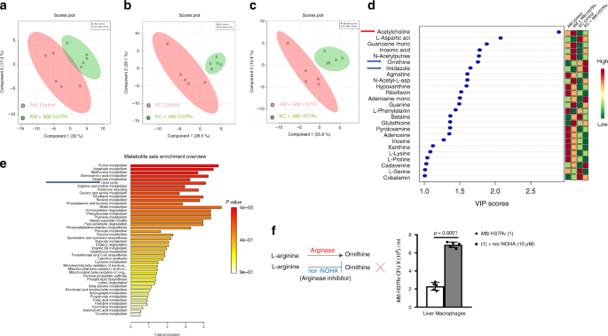Fig. 4: Metabolic profiles ofMtb-infected AMs and KCs. AMs and KCs from C57BL/6 mice were isolated and infected withMtbH37Rv. After 72 h, cell lysates were analyzed using LC-MS. A representative score plot of the partial least squares discriminant analysis (PLS-DA) was generated using MetaboAnalyst. PLS-DA models were validated using R2and Q2based on LOOCV (leave one out cross-validation); the four-component model was selected as the optimized model withR2= 0.95 andQ2= 0.58. The significance of the model was demonstrated by a permutation test with 100 testing iterations using a separation distance ofp< 0.01.aAMs control (red); AMsMtbH37Rv (green).bKCs control (red); KCsMtbH37Rv (green).cAMsMtbH37Rv (red); KCsMtbH37Rv (green).dRepresentation of 25 metabolites with VIP (variable importance of projection) scores greater than 1.0 based on PLS-DA considered significant. On the extreme right, red and green indicates high and low levels of metabolites, respectively.eQuantitative metabolite sets enrichment overview using metabolite set enrichment analysis (MSEA) with the fold change showing the metabolic pathways of 25 metabolites selected based on their VIP scores greater than 1. The arrow indicates upregulated metabolites and pathways inMtbH37Rv-infected KCs.fKCs from C57BL/6 mice were isolated and infected withMtbH37Rv at an MOI of 1:2.5 (1 AM and 2.5Mtb). At 2 h post-infection, nor-NOHA were added at indicated concentrations. Intracellular CFUs were demonstrated 5 days post-infection. Statistical analysis was performed with paired two-tailed t test and presented as mean ± SD. Data shown are representative of five independent experiments. Subsequently, the slides were washed thoroughly 3 × 5 min with PBS. Then, the tissue sections were stained with the respective secondary antibodies at 1:500 dilutions (v/v), washed again with PBS for 3 × 5 min, and mounted with fluoroshield mounting medium with DAPI. The mounted slides were then examined and analyzed under a laser-scanning confocal microscope (Zeiss LSM 510 Meta laser-scanning confocal microscope). Statistical analysis Data analyses were performed using Graph Pad Prism 7.0 (GraphPad Software, Inc., La Jolla, CA). Real-time PCR and CFU data are expressed as the mean ± SD. For normally distributed data, comparisons between groups were performed using a paired or unpaired t-test and ANOVA, as appropriate. Differences were considered statistically significant with a p value < 0.05. Metabolomics data analysis was carried out using the Metaboanalyst 3.0 software. 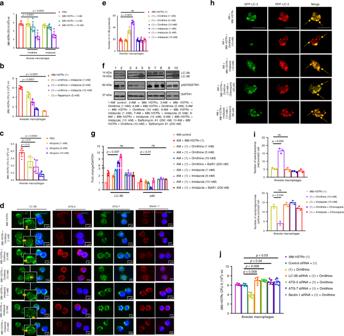Fig. 5: Ornithine, imidazole and atropine affectMtbgrowth. AMs were infected withMtbH37Rv. At 2 h post-infection, ornithine and imidazole alone or in combination were added alongside atropine. Intracellular CFUs were demonstrated after 5 days post-infection.aOrnithine and imidazole alone,bin combination of both,catropine.p< 0.0181,p< 0.0112.n= 5 experiments each.dA representative micrograph of LC3-B, ATG-7, ATG-5 and Beclin-1 in AMs and KCs. Blue: DAPI; green: LC-3B and ATG-7; red: ATG-5 and Beclin-1. Images of multiple fields at 63× magnification were taken with oil immersion.eThe number of LC-3B puncta relative to the cell area (10 cells per condition) was quantified using ImageJ. Data shown are representative of five independent experiments.fTotal protein was extracted and western blotting was performed. A representative blot depicting the levels of LC-3 and p62/SQSTM1 in the control andMtb-infected macrophages followed by treatment with ornithine and imidazole is shown. GAPDH was used as a loading control.gNormalized fold intensities of LC-3B and p62 levels inMtb-infected and ornithine or imidazole treated macrophages compared with the levels in the uninfected control.p< 0.0072,p< 0.019, ns not significant.n= 3 experiments.hAlveolar macrophages were labeled with an autophagy sensor expressing RFP-GFP-LC3B for 48 h. Macrophages were then infected withMtbfollowed by treatment with ornithine or imidazole for 72 h. Cells were fixed, and LC-3 was analyzed by confocal microscopy. Scale bars: 5 µm.iQuantification of the number of LC-3B positive autophagosomes (yellow fluorescence) and autolysosomes (red fluorescence) in control andMtb-infected macrophages treated with ornithine and imidazole.p< 0.0041,p< 0.0034.n= 3 experiments.jAMs from C57BL/6 mice were isolated and transfected with the siRNAs targeting LC-3B, ATG-5, ATG-7 and Beclin-1 or with control siRNA, infected withMtband then treated with 10 mM ornithine. After 5 days, CFUs were counted.p< 0.0097,p< 0.0067,p< 0.046,p< 0.0327.n= 5 experiments. Data are presented as the mean ± SD using paired two-tailed t test. Partial least squares discriminant analysis (PLS-DA) was performed as a supervised method to identify important variables with discriminative power. PLS-DA models were validated based on the multiple correlation coefficient ( R 2 ) and cross-validated R 2 ( Q 2 ) by cross-validation and permutation tests by applying 100 iterations ( p > 0.001). The significance of the biomarkers was ranked using the variable importance in projection (VIP) score (>1) from the PLS-DA model. 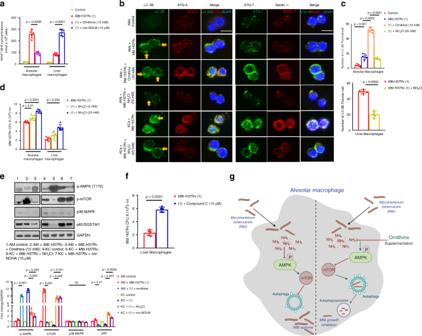Fig. 6: Ornithine limits ammonia and activates AMPK. AMs and KCs from C57BL/6 mice were isolated and infected withMtbH37Rv at an MOI of 1:2.5. After 72 h.aNH4+/NH3levels were measured in the cell lysates treated with ornithine or nor-NOHA (arginase inhibitor) by spectrophotometric analysis at 570 nm with extrapolation from the standard curve and expressed in nmol (mean ± SD). Data are representatives of five independent experiments.bA representative micrograph of LC3-B, ATG-7, ATG-5 and Beclin-1 in AMs treated with ornithine or NH4Cl and KCs treated with NH4Cl at respective concentrations. Blue: DAPI; green: LC-3B and ATG-7; red: ATG-5 and Beclin-1. Scale bar: 5 μm. Images of multiple fields at 63× magnification were taken with oil immersion.cThe number of LC-3B puncta relative to the cell area (10 cells per condition) was quantified using ImageJ.p< 0.0012.dAt 2 h post-infection, NH4Cl was added at the indicated concentrations. Intracellular CFUs were demonstrated after 5 days of infection.p< 0.0195,p< 0.0042.n= 5 experiments.eTotal protein was extracted from the above cells and western blotting was performed. A representative blot depicting the levels of p-AMPK, p-mTOR, p38 MAPK, LC-3 and p62/SQSTM1 in the control, ornithine or NH4Cl treated andMtbH37Rv-infected macrophages is shown. Normalized fold intensities of p-AMPK,p< 0.0013,p< 0.0032,p< 0.0051; p-mTOR,p< 0.0017,p< 0.0027,p< 0.0018; p38 MAPK, ns not significant; and p62 levelsp< 0.0191,p< 0.0072 inMtb-infected and ornithine or NH4Cl treated macrophages compared with the levels in the uninfected control.n= 3 experiments.fAt 2 h post-infection, ornithine and compound C were added at indicated concentrations. Intracellular CFUs were demonstrated after 5 days of infection.n= 5 experiments. Data are presented as the mean ± SD and analyzed using paired two-tailed t test.gSchematic representation of ornithine restrictingMtbgrowth in AMs. Red color indicates inhibitory line and green arrows indicates activation. 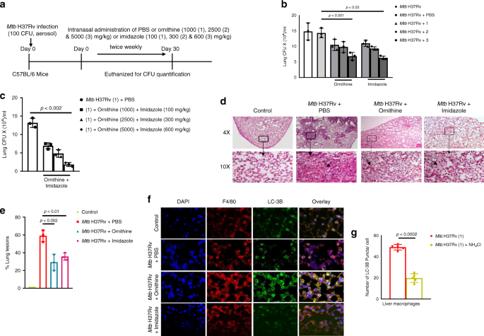Fig. 7: Ornithine and imidazole restrictMtbgrowth in the lungs. C57BL/6 mice were infected with 100 CFU of aerosolizedMtbH37Rv, and then treated with ornithine and imidazole at varying concentrations.aSchematic representation ofMtbinfection and intranasal delivery of the compounds.b,cBacterial burden in the lungs measured after one-month post-infection and post-treatment. Data are representative of three independent experiments (n= 5 mice per group). Data are expressed as the mean ± SD.p< 0.0015.cMtb-infected mice were treated in combination of ornithine/imidazole, one group treated with 1000/100 mg/kg, other as 2500/300 mg/kg and last group as 5000/600 mg/kg.p< 0.0029.d–fAt one-month post-infection and post-treatment, the lungs of the uninfected control,Mtb-infected, ornithine or imidazole treated mice were isolated and formalin-fixed. Paraffin-embedded tissue sections were prepared, and hematoxylin and eosin staining was performed. Inflamed lung areas were compared among the groups.dA representative figure is shown.ePercentage of the lung lesions was calculated.p< 0.0024,p< 0.0192.fParaffin-embedded lung tissue sections were analyzed by confocal microscopy to evaluate LC-3B (green), F4/80 (far-red) staining as well as their colocalization. Scale bar: 10 μm. A representative micrograph of LC-3B in lungs is shown. Images of multiple fields at 63× magnification were taken with oil immersion.gThe immunofluorescence intensity (A.U.) of LC-3B are shown. Data are representative of three independent experiments. Five mice per group were used for each independent experiment.p< 0.0013. Statistical analysis was performed using paired two-tailed t test and data are represented as the mean ± SD. Metabolite set enrichment analysis (MSEA) was performed to identify the biologically meaningful patterns that were significantly enriched in selected and additional representative metabolites. Reporting summary Further information on research design is available in the Nature Research Reporting Summary linked to this article.